Calcium-dependent FAK/CREB/TNNC1 signalling mediates the effect of stromal MFAP5 on ovarian cancer metastatic potential Ovarian cancer is the most lethal gynaecologic malignancy in the United States, and advanced serous ovarian adenocarcinoma is responsible for most ovarian cancer deaths. However, the stroma-derived molecular determinants that modulate patient survival are yet to be characterized. Here we identify a stromal gene signature for advanced high-grade serous ovarian cancer using microdissected stromal ovarian tumour samples and find that stromal microfibrillar-associated protein 5 ( MFAP5 ) is a prognostic marker for poor survival. Further functional studies reveal that FAK/CREB/TNNC1 signalling pathways mediate the effect of MFAP5 on ovarian cancer cell motility and invasion potential. Targeting stromal MFAP5 using MFAP5 -specific siRNA encapsulated in chitosan nanoparticles significantly decreases ovarian tumour growth and metastasis in vivo , suggesting that it may be a new modality of ovarian cancer treatment. Ovarian cancer is the fifth most common cancer in women in the United States. Epithelial ovarian cancer is the most common subtype and is highly lethal. Researchers estimated that 21,980 new cases of ovarian cancer would be diagnosed and 14,270 patients would die of ovarian cancer in the United States in 2014 (ref. 1 ). Although this disease is initially sensitive to platinum- and taxane-based chemotherapy following debulking surgery, most patients experience recurrence within 12–24 months and die of progressively chemotherapy-resistant disease. Markers that can be used to predict chemotherapy response and survival are yet to be thoroughly explored. A critically important yet often overlooked component of tumour progression is the tumour microenvironment, which is composed of fibroblasts, extracellular matrix proteins, endothelial cells and lymphocytic infiltrates. The tumour microenvironment can directly affect cell growth, migration and differentiation via secreted proteins, cell–cell interactions and matrix remodelling [2] . It also promotes tumour initiation via transformation of normal epithelial cells and facilitates the progression of malignant cells, thereby presenting a unique challenge to diagnosing, understanding and treating cancer. Previous large-scale transcriptome profiling studies, including The Cancer Genome Atlas, identified prognostic gene signatures for advanced high-grade serous ovarian cancer (HGSC) using bulk or microdissected ovarian tumour samples [3] , [4] , [5] , [6] . However, large-scale transcriptome profiles generated using the stromal component of ovarian tumours are lacking, and the prognostic significance of stromal gene expression in ovarian cancer cells remains largely unknown. In the present study, we sought to determine the stromal signature of HGSC and identify specific genes that are associated with patient survival using microdissected tumour samples. We used a whole-genome oligonucleotide array to perform transcriptome profiling of the fibroblastic stromal components microdissected from a series of HGSC patients (informed consent was obtained from all subjects under protocols approved by the MD Anderson Institutional Review Board) to identify a transcriptome signature for ovarian cancer-associated fibroblasts (CAFs). Furthermore, we functionally characterized microfibrillar-associated protein 5, MFAP5 (Previously known as microfibril-associated glycoprotein 2, MAGP2), a gene that we identified in the gene signature, determined its prognostic significance and evaluated the molecular mechanism that mediates its effect on ovarian cancer cell motility and invasion potential. Accession codes: Data files from the transcriptome profiling analysis were deposited in the Gene Expression Omnibus (GEO; National Center for Biotechnology Information, Bethesda, MD, USA). Transcriptome profiling data for microdissected ovarian tissue samples were assigned the GEO accession number GES40595 , and microarray data for MFAP5-treated OVCA432 cells were assigned the GEO accession number GES40643 . Ovarian CAFs express MFAP5 at high levels The stromal microenvironment is known to provide a niche that supports tumour growth [2] . To identify mediators produced by the stromal microenvironment that support ovarian tumour growth, we performed transcriptome profiling of microdissected stromal and epithelial components of ovarian tumour tissues. Among the differentially expressed genes, we identified 19 upregulated secretory protein-coding genes in the stromal component of HGSC samples ( Fig. 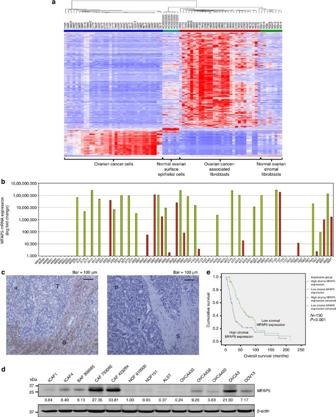Figure 1: Identification of MFAP5 as one of the most highly overexpressed proteins in ovarian CAFs with clinical significance. (a) Heat map showing 819 significantly differentially expressed genes in microdissected CAFs and ovarian epithelial tumour samples obtained from 33 patients, normal stromal fibroblasts obtained from eight normal ovaries and six normal ovarian surface epithelial tissue samples. (b) Quantitative RT–PCR analysis of RNA isolated from microdissected normal ovarian cortical fibroblasts, and the stromal fibroblastic (S: green bars) and epithelial (T: red bars) components from the same patients are shown. Normal fibroblasts did not have MFAP5 expression. Cancer stromal fibroblasts had significantly higher levels ofMFAP5expression than did those in the epithelial components. (c) Immunolocalization of MFAP5 in advanced HGSC samples with high (a) and low (b) levels of MFAP5 expression in the cancer stroma. S, cancer stroma; T, epithelial component. Bar=100 μm. (d) Western blot analysis demonstrating higher levels of MFAP5 expression in CAFs than in NOFs and ovarian cancer cells. Relative normalized protein expression levels are shown. (e) Immunolocalization of MFAP5 was performed on 130 advanced HGSC tissue samples to determine the clinical relevance of stromal MFAP5 expression and HGSC patient survival. Kaplan–Meier analysis revealed that low stromal MFAP5 expression was significantly associated with a longer overall survival duration than patients who have high stromal MFAP5 expression (P<0.001; log-rank test). Patients with high (above the median) and low (at or below the median) stromal MFAP5 expression levels had a median overall survival duration of 24 and 54 months, respectively. 1a and Table 1 ). MFAP5 , which we have shown to be amplified and overexpressed in a subset of ovarian cancer cells [6] , was selected for further validation. Validation with quantitative real-time PCR revealed significantly higher levels of MFAP5 mRNA expression in the cancer stroma than the epithelial components and normal ovarian stroma ( Fig. 1b ). Immunohistochemistry also revealed a higher level of MFAP5 protein expression in the cancer-associated stroma, particularly in CAFs, than in normal ovarian fibroblasts (NOFs) and ovarian cancer cells ( Fig. 1c ). Western blot analysis confirmed a higher endogenous level of MFAP5 in ovarian CAFs when compared with normal fibroblasts and ovarian cancer cell lines ( Fig. 1d ). Figure 1: Identification of MFAP5 as one of the most highly overexpressed proteins in ovarian CAFs with clinical significance. ( a ) Heat map showing 819 significantly differentially expressed genes in microdissected CAFs and ovarian epithelial tumour samples obtained from 33 patients, normal stromal fibroblasts obtained from eight normal ovaries and six normal ovarian surface epithelial tissue samples. ( b ) Quantitative RT–PCR analysis of RNA isolated from microdissected normal ovarian cortical fibroblasts, and the stromal fibroblastic (S: green bars) and epithelial (T: red bars) components from the same patients are shown. Normal fibroblasts did not have MFAP5 expression. Cancer stromal fibroblasts had significantly higher levels of MFAP5 expression than did those in the epithelial components. ( c ) Immunolocalization of MFAP5 in advanced HGSC samples with high ( a ) and low ( b ) levels of MFAP5 expression in the cancer stroma. S, cancer stroma; T, epithelial component. Bar=100 μm. ( d ) Western blot analysis demonstrating higher levels of MFAP5 expression in CAFs than in NOFs and ovarian cancer cells. Relative normalized protein expression levels are shown. ( e ) Immunolocalization of MFAP5 was performed on 130 advanced HGSC tissue samples to determine the clinical relevance of stromal MFAP5 expression and HGSC patient survival. Kaplan–Meier analysis revealed that low stromal MFAP5 expression was significantly associated with a longer overall survival duration than patients who have high stromal MFAP5 expression ( P <0.001; log-rank test). Patients with high (above the median) and low (at or below the median) stromal MFAP5 expression levels had a median overall survival duration of 24 and 54 months, respectively. Full size image Table 1 Secretory proteins upregulated in CAFs compared with HOSE, NOFs and ovarian cancer epithelia. Full size table Stromal MFAP5 overexpression predicts poor survival To determine the clinical significance of stromal MFAP5 expression, we performed MFAP5 immunolocalization on 130 advanced HGSC samples. Kaplan–Meier analysis showed that high stromal MFAP5 expression is significantly associated with poor clinical outcomes ( P <0.001; log-rank test; Fig. 1e ). Cox regression analysis with adjustment for age and debulking status confirmed the prognostic significance of stromal MFAP5 expression (hazard ratio, 2.603; P =0.001). Stromal MFAP5 stimulates cancer cell motility and invasion Previous studies by our group revealed that MFAP5 could exert its effect on cancer cells in an autocrine manner via binding of its RGD domain to αVβ3 integrin. To determine CAF-derived MFAP5’s role in ovarian cancer progression, CAFs expressing high levels of MFAP5 were co-cultured with A224 and ALST ovarian cancer cells, which have undetectable levels of endogenous MFAP5 and high levels of αVβ3 integrin expression ( Supplementary Fig. 1 ). Experimental results demonstrated that anti-MFAP5 and anti-αVβ3 integrin antibodies attenuated the stimulatory effect of MFAP5 on cancer cell motility ( P <0.001; two-tailed Student’s t -test; Fig. 2a ). 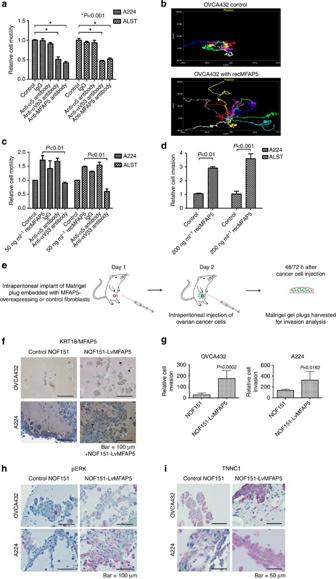Figure 2: Stromal MFAP5-induced ovarian cancer cell motility and invasion potentialin vitroandin vivo. (a) Relative motility of ovarian cancer cells when co-cultured with CAF793092 primary ovarian CAFs in the presence of different antibodies was studied. Control IgG and anti-α5 antibodies did not affect cancer cell motility, while anti-αVβ3 and anti-MFAP5 antibodies attenuated cancer cell motility in the co-culture system (mean±s.d. of three independent experiments;P<0.001; two-tailed Student’st-test). (b) A series of images obtained from the treatment of OVCA432 cells with recombinant MFAP5 protein in an temperature-controlled imaging chamber for 48 h was analysed using the MetaMorph software programme for tracking of the movement of individual cells. Presence of exogenous MFAP5-enhanced OVCA432 cell motility. (c) Relative motility of cancer cells was evaluated after treatment with recombinant MFAP5 in the presence of control IgG, anti-α5 or anti-αVβ3 antibodies compared with antibody-free controls; the presence of anti-αVβ3 antibodies abrogated MFAP5-induced cell motility (mean±s.d. of three independent experiments;P<0.01; two-tailed Student’st-test). (d) Invasion assay using Matrigel invasion chamber showed that recombinant MFAP5-enhanced ovarian cancer cell invasiveness (mean±s.d. of three independent experiments;P<0.001; two-tailed Student’st-test). (e) A schematic diagram showing the procedures of using intraperitoneally implanted Matrigel plugs to evaluate the effects of MFAP5 on invasion potential of ovarian cancer cells. (f,g) Immunolocalization of MFAP5 (red signal) and cytokeratin 18 (brown signal) on paraffin section Matrigel plugs collected from the peritoneal cavities of mice; Bar=100 μm. The invaded cancer cells with cytokeratin 18 staining were quantified using the Image-Pro Plus software programme (mean±s.d.;n=10 Matrigel plugs per treatment group for each cell line;P=0.0002 and 0.0162 for OVCA432 and A224 cells, respectively; Mann–WhitneyU-test). Staining for MFAP5 showed that MFAP5-positive cells were found only in Matrigel plugs embedded with MFAP5-overexpressing fibroblasts, suggesting that stromal MFAP5 promoted ovarian cancer cell invasion into the plugs implanted. (h,i) Immunolocalization of p-ERK1/2 and troponin C in paraffin sections of Matrigel plugs collected from the peritoneal cavities of mice demonstrating that the effects of stromal MFAP5 on cancer cell motility and invasion potential were mediated by the upregulation of p-ERK1/2 and troponin C expression; bar=100 and 50 μm, respectively. Figure 2: Stromal MFAP5-induced ovarian cancer cell motility and invasion potential in vitro and in vivo . ( a ) Relative motility of ovarian cancer cells when co-cultured with CAF793092 primary ovarian CAFs in the presence of different antibodies was studied. Control IgG and anti-α5 antibodies did not affect cancer cell motility, while anti-αVβ3 and anti-MFAP5 antibodies attenuated cancer cell motility in the co-culture system (mean±s.d. of three independent experiments; P <0.001; two-tailed Student’s t -test). ( b ) A series of images obtained from the treatment of OVCA432 cells with recombinant MFAP5 protein in an temperature-controlled imaging chamber for 48 h was analysed using the MetaMorph software programme for tracking of the movement of individual cells. Presence of exogenous MFAP5-enhanced OVCA432 cell motility. ( c ) Relative motility of cancer cells was evaluated after treatment with recombinant MFAP5 in the presence of control IgG, anti-α5 or anti-αVβ3 antibodies compared with antibody-free controls; the presence of anti-αVβ3 antibodies abrogated MFAP5-induced cell motility (mean±s.d. of three independent experiments; P <0.01; two-tailed Student’s t -test). ( d ) Invasion assay using Matrigel invasion chamber showed that recombinant MFAP5-enhanced ovarian cancer cell invasiveness (mean±s.d. of three independent experiments; P <0.001; two-tailed Student’s t -test). ( e ) A schematic diagram showing the procedures of using intraperitoneally implanted Matrigel plugs to evaluate the effects of MFAP5 on invasion potential of ovarian cancer cells. ( f , g ) Immunolocalization of MFAP5 (red signal) and cytokeratin 18 (brown signal) on paraffin section Matrigel plugs collected from the peritoneal cavities of mice; Bar=100 μm. The invaded cancer cells with cytokeratin 18 staining were quantified using the Image-Pro Plus software programme (mean±s.d. ; n =10 Matrigel plugs per treatment group for each cell line; P =0.0002 and 0.0162 for OVCA432 and A224 cells, respectively; Mann–Whitney U -test). Staining for MFAP5 showed that MFAP5-positive cells were found only in Matrigel plugs embedded with MFAP5-overexpressing fibroblasts, suggesting that stromal MFAP5 promoted ovarian cancer cell invasion into the plugs implanted. ( h , i ) Immunolocalization of p-ERK1/2 and troponin C in paraffin sections of Matrigel plugs collected from the peritoneal cavities of mice demonstrating that the effects of stromal MFAP5 on cancer cell motility and invasion potential were mediated by the upregulation of p-ERK1/2 and troponin C expression; bar=100 and 50 μm, respectively. Full size image Real-time imaging of the HGSC cell line OVCA432 treated with purified recombinant MFAP5 protein (recMFAP5) revealed that exogenous recMFAP5 increased OVCA432 cell motility ( Fig. 2b ). To further validate the motility-stimulating effects of exogenous MFAP5, Boyden chamber-based motility assays were performed on A224 and ALST cell lines. Increased migrated cells were observed in both recMFAP5-treated cell lines. Presence of anti-αVβ3 antibody attenuated the stimulatory effect of MFAP5 on cell motility ( P <0.01; two-tailed Student’s t -test) ( Fig. 2c ). Data from the co-culture studies and exogenous MFAP5 treatment confirmed that the stimulatory effect of MFAP5 on ovarian cancer cell motility was mediated by its binding to the αVβ3 integrin receptor. In addition, A224 and ALST cells seeded on Matrigel matrix with recMFAP5 resulted in three times the number of cells invaded through the matrix when compared with the control ( Fig. 2d ), suggesting that MFAP5 also stimulated the invasion potential of the ovarian cancer cells. MFAP5 stimulates cancer cell motility and invasion in vivo To determine the effects of exogenous MFAP5 on ovarian tumour growth in vivo , a MFAP5-overexpressing NOF line was generated. Overexpression of MFAP5 was confirmed with western blot analysis ( Supplementary Fig. 2A ). Cell proliferation assay was performed to confirm similar proliferation rates in MFAP5-overexpressing and control cells ( Supplementary Fig. 2B ). For the mouse study, fibroblasts-embedded Matrigel plugs were intraperitoneally implanted into nude mice followed by cancer cell injection ( Fig. 2e ). Matrigel plugs harvested were double-stained for cytokeratin 18 and MFAP5. Results showed that more cancer cells were found in Matrigel plugs embedded with MFAP5-overexpressing fibroblasts than those embedded with control fibroblasts ( Fig. 2f,g ), suggesting that stromal MFAP5 promoted ovarian cancer cell migration and invasion into the Matrigel plugs. In vivo Mfap5 silencing reduces tumour progression To evaluate the effect of stromal MFAP5 silencing on ovarian cancer metastasis, we silenced murine stromal Mfap5 in an orthotopic model of ovarian carcinoma [7] , [8] by intravenous injection of Mfap5 -specific short interfering RNAs (siRNAs) incorporated into chitosan nanoparticles (CH-NP; Fig. 3a ). The efficacy of these siRNA sequences on Mfap5 silencing was evaluated in murine fibroblasts using both quantitative RT-PCR and western blot analyses ( Supplementary Fig. 3A ). One week after initial cancer cell injection, two Mfap5 -targeting siRNAs and a nontargeting sequence were packaged in CH-NP and delivered via tail vein injection to luciferase-labelled cancer cell-bearing nude mice twice a week throughout the course of the experiment. Markedly lower luciferase activity was detected in Mfap5 knockdown groups compared with the control group at week 6 ( Fig. 3b ). At the end point of the study, necropsy revealed amelioration of cancer metastasis in the stromal Mfap5 -silenced groups when compared with the control group ( Fig. 3c ). Mfap5 siRNAs/CH-NP resulted in a significant decrease in the number of metastatic tumour nodules found at mesentery, omentum, peritoneum, diaphragm, liver and spleen ( P <0.001; Mann–Whitney U -test), tumour weight ( P <0.001; Mann–Whitney U -test) and ascite volume ( P <0.001; Mann–Whitney U -test; Fig. 3d ), suggesting that stromal Mfap5 silencing inhibited ovarian tumour growth and metastatic spread. Primary tumour burden was quantified by measuring the primary tumour area in the ovaries using images of haematoxylin and eosine tissue sections prepared from tumours harvested from the three treatment groups. Similar primary tumour burdens were observed in the control and Mfap5-targeted animal groups suggesting that reduced metastasis observed in the MFAP5-targeting siRNA treatment group is the result from reduced cancer cell motility and invasive potential instead of reduced primary tumour burden ( Fig. 3e ). Immunostaining was performed on paraffin sections of tumour tissue harvested to validate in vivo silencing of murine stromal Mfap5 ( Fig. 3f ). 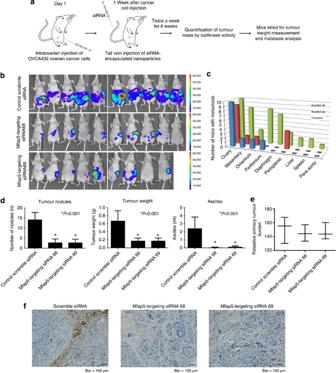Figure 3:In vivostromal Mfap5 silencing reduced ovarian tumour growth and metastasis. (a) A schematic diagram showing the procedures of using intraovarian tumour injection model to evaluate the effects of MFAP5 on invasion and metastatic potential of ovarian cancer cells. (b) Luciferase-labelled ovarian cancer cells were injected into left ovary of nude mice and luminescence was measured at week 6. Luciferase activities were significantly weaker in stromalMfap5-silenced groups when compared with the control siRNA groups (N=9–10 per treatment group). (c) Reduced metastatic spread of cancer cells within the abdominal cavity was observed in theMfap5siRNA-encapsulated chitosan nanoparticle-treated groups when compared with the control group. (d) Significantly reduced number of metastatic tumour nodules, tumour weight and ascites volume were observed in the Mfap5 knockdown groups when compared with the control siRNA group after necropsy (mean±s.d.;n=9–10 per treatment group;P<0.001; Mann–WhitneyU-test). (e) Primary tumour burden was quantified by measuring the primary tumour area in the ovaries using images of haematoxylin and eosine tissue sections prepared from tumours harvested from the control scramble siRNA treatment groups and two Mfap5-targeting siRNA treatment groups. Similar primary tumour burdens were observed in the control and Mfap5-targeted animal groups based on Mann–WhitneyU-tests. (f) Tumour tissues were fixed in formalin and embedded with paraffin followed by immunolocalization of Mfap5 to confirm the successful knockdown of stromal Mfap5 expression. S, Stroma; T, Tumour; Bar=100 μm. Figure 3: In vivo stromal Mfap5 silencing reduced ovarian tumour growth and metastasis. ( a ) A schematic diagram showing the procedures of using intraovarian tumour injection model to evaluate the effects of MFAP5 on invasion and metastatic potential of ovarian cancer cells. ( b ) Luciferase-labelled ovarian cancer cells were injected into left ovary of nude mice and luminescence was measured at week 6. Luciferase activities were significantly weaker in stromal Mfap5 -silenced groups when compared with the control siRNA groups ( N =9–10 per treatment group). ( c ) Reduced metastatic spread of cancer cells within the abdominal cavity was observed in the Mfap5 siRNA-encapsulated chitosan nanoparticle-treated groups when compared with the control group. ( d ) Significantly reduced number of metastatic tumour nodules, tumour weight and ascites volume were observed in the Mfap5 knockdown groups when compared with the control siRNA group after necropsy (mean±s.d. ; n =9–10 per treatment group; P <0.001; Mann–Whitney U -test). ( e ) Primary tumour burden was quantified by measuring the primary tumour area in the ovaries using images of haematoxylin and eosine tissue sections prepared from tumours harvested from the control scramble siRNA treatment groups and two Mfap5-targeting siRNA treatment groups. Similar primary tumour burdens were observed in the control and Mfap5-targeted animal groups based on Mann–Whitney U -tests. ( f ) Tumour tissues were fixed in formalin and embedded with paraffin followed by immunolocalization of Mfap5 to confirm the successful knockdown of stromal Mfap5 expression. S, Stroma; T, Tumour; Bar=100 μm. Full size image MFAP5 upregulates TNNC1 via the Ca 2+ -dependent pathway Transcriptome profiling on MFAP5-treated and -untreated OVCA432 cells followed by pathway analysis identified a set of upregulated motility-promoting genes associated with calcium signalling in recMFAP5-treated cells ( Fig. 4a,b ). Troponin C type 1 ( TNNC1 ) was chosen for further studies. TNNC1 contains a calcium-binding subunit and facilitates the interaction between actin and myosin in skeletal and cardiac muscle cells and the formation of stress fibres, suggesting that it may play a key role in mediating MFAP5’s stimulatory effect on ovarian cancer cell motility. We performed quantitative RT–PCR analysis on five MFAP5-treated ovarian cancer cell lines and observed a significant increase in TNNC1 expression in all of them ( Fig. 4c ). Results of motility assays demonstrated that silencing of TNNC1 by a validated TNNC1-targeting siRNA ( Supplementary Fig. 3B,C ) abolished MFAP5’s stimulatory effect on A224 and ALST cell motility ( Fig. 4d ), suggesting that TNNC1 is the effector protein for MFAP5-enhanced cancer cell motility. In addition, F-actin staining showed that recMFAP5 treatment led to an F-actin cytoskeleton with increased density and organization in ovarian cancer cells ( Fig. 4e ), but that these effects were abrogated in TNNC1 siRNA-transfected cells ( Supplementary Fig. 4 ) suggested that MFAP5 stimulated cell motility via induction of TNNC1 expression and F-actin cytoskeleton reorganization. 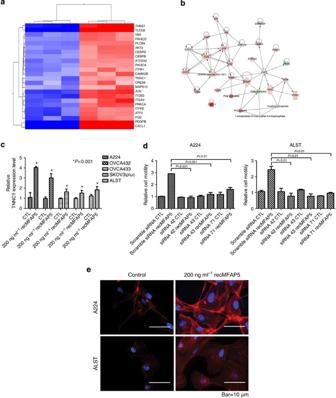Figure 4: Contribution of calcium-dependent signalling pathway activation, TNNC1 overexpression and F-actin cytoskeleton reorganization to MFAP5-stimulated ovarian cancer cell motility. (a) Heat map of motility-promoting genes associated with calcium signalling whose expression was upregulated in MFAP5-treated OVCA432 cells. (b) Interacting network of motility-promoting and calcium signalling-related genes whose expression was upregulated at least 1.5-fold in MFAP5-treated OVCA432 cells created using the Ingenuity Pathway Analysis software programme (Ingenuity Systems, Redwood City, CA, USA). (c) Upregulation ofTNNC1mRNA expression in five serous ovarian cancer cell lines after MFAP5 treatment (mean±s.d. of three independent experiments;P<0.001; two-tailed Student’st-test). (d) Abrogation of MFAP5’s stimulatory effect on ovarian cancer cell motility by knockdown of TNNC1 expression usingTNNC1-targeting siRNAs and a scrambled nontargeting siRNA as control (mean±s.d. of three independent experiments; two-tailed Student’st-test). (e) MFAP5-induced F-actin rearrangement and activated stress fibre formation in A224 and ALST cells; bar=10 μm. Figure 4: Contribution of calcium-dependent signalling pathway activation, TNNC1 overexpression and F-actin cytoskeleton reorganization to MFAP5-stimulated ovarian cancer cell motility. ( a ) Heat map of motility-promoting genes associated with calcium signalling whose expression was upregulated in MFAP5-treated OVCA432 cells. ( b ) Interacting network of motility-promoting and calcium signalling-related genes whose expression was upregulated at least 1.5-fold in MFAP5-treated OVCA432 cells created using the Ingenuity Pathway Analysis software programme (Ingenuity Systems, Redwood City, CA, USA). ( c ) Upregulation of TNNC1 mRNA expression in five serous ovarian cancer cell lines after MFAP5 treatment (mean±s.d. of three independent experiments; P <0.001; two-tailed Student’s t -test). ( d ) Abrogation of MFAP5’s stimulatory effect on ovarian cancer cell motility by knockdown of TNNC1 expression using TNNC1 -targeting siRNAs and a scrambled nontargeting siRNA as control (mean±s.d. of three independent experiments; two-tailed Student’s t -test). ( e ) MFAP5-induced F-actin rearrangement and activated stress fibre formation in A224 and ALST cells; bar=10 μm. Full size image MFAP5 enhances Ca 2+ mobilization and cell traction force Transcriptome profiling and pathway analysis data suggest that cytosolic calcium mobilization is integral to MFAP5’s effect on ovarian cancer motility. The observations that MFAP5’s motility stimulatory effect was attenuated and F-actin-reorganizing effect was abrogated in calcium chelator BAPTA/AM-preloaded cancer cells ( Fig. 5a,b ), suggesting that calcium signalling is involved in modulating MFAP5’s functions. Using the calcium dye Fluo-4 AM and confocal fluorescence microscopy, we observed that exogenous MFAP5 mobilized intracellular Ca 2+ in A224 and ALST cells ( Fig. 5c ). Further evaluation on the mechanisms involved in calcium mobilization in ALST cells showed that treatment with the L-type Ca 2+ channel blocker nifedipine attenuated but did not abolish MFAP5-induced calcium mobilization ( Supplementary Fig. 5A ). The channel opener BAYK8644 triggered calcium mobilization in ALST cells ( Supplementary Fig. 5B ), suggesting that MFAP5 induced exogenous Ca 2+ entry. In addition, treatment with the IP 3 receptor inhibitor xestospongin C but not the ryanodine receptor blocker attenuated MFAP5-induced calcium mobilization, suggesting that IP 3 -sensitive Ca 2+ stores are mobilized by MFAP5 ( Supplementary Fig. 5C,D ). As IP 3 -sensitive Ca 2+ store depletion can trigger store-operated Ca 2+ entry and is a common entry pathway in nonexcitable cells, we confirmed that an exogenous Ca 2+ entry mechanism resembling store-operated calcium entry was present in ALST cells ( Supplementary Fig. 5E ). 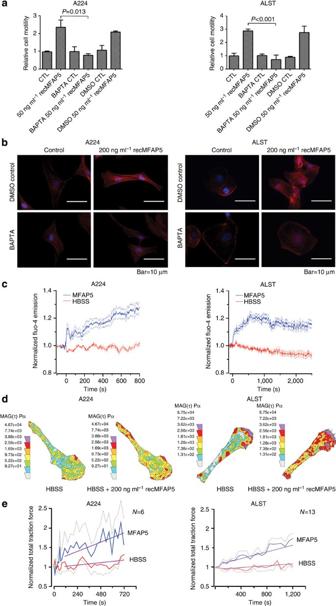Figure 5: Effects of MFAP5 on motility are mediated via calcium mobilization and increasing traction force in ovarian cancer cells. (a) Attenuation of the stimulatory effect of MFAP5 on ovarian cancer cell motility by the cell-permeant calcium chelator BAPTA/AM but not the solvent control dimethylsulphoxide (mean±s.d. of three independent experiments;P=0.013 and <0.001 for A224 and ALST cells, respectively; two-tailed Student’st-test). (b) Abrogation of activated stress fibre formation and actin reorganization in A224 and ALST cells pretreated with BAPTA/AM but not those pretreated with DMSO; bar=10 μm. (c) The mean normalized time course of Ca2+mobilization in A224 and ALST cells induced by MFAP5. HBSS containing MFAP5 or the HBSS alone was added to the bath of cells att=0 (mean±s.e.m. of four independent experiments for each treatment group). (d) Cell traction force maps of A224 and ALST cells before and after exposure to MFAP5. (e) The normalized total traction force exerted by A224 and ALST cells induced by MFAP5. Dotted grey lines are SEM. Only one side of SEM is shown. Purple lines are regression lines. HBSS containing MFAP5 or HBSS alone was added to the bath of cells att=120 s. MFAP5 significantly increases the slope of regression line compared with that of HBSS in both cell lines (P<0.05; two-tailed Student’st-test).N=number of cells used for the normalized time course. Figure 5: Effects of MFAP5 on motility are mediated via calcium mobilization and increasing traction force in ovarian cancer cells. ( a ) Attenuation of the stimulatory effect of MFAP5 on ovarian cancer cell motility by the cell-permeant calcium chelator BAPTA/AM but not the solvent control dimethylsulphoxide (mean±s.d. of three independent experiments; P =0.013 and <0.001 for A224 and ALST cells, respectively; two-tailed Student’s t -test). ( b ) Abrogation of activated stress fibre formation and actin reorganization in A224 and ALST cells pretreated with BAPTA/AM but not those pretreated with DMSO; bar=10 μm. ( c ) The mean normalized time course of Ca 2+ mobilization in A224 and ALST cells induced by MFAP5. HBSS containing MFAP5 or the HBSS alone was added to the bath of cells at t =0 (mean±s.e.m. of four independent experiments for each treatment group). ( d ) Cell traction force maps of A224 and ALST cells before and after exposure to MFAP5. ( e ) The normalized total traction force exerted by A224 and ALST cells induced by MFAP5. Dotted grey lines are SEM. Only one side of SEM is shown. Purple lines are regression lines. HBSS containing MFAP5 or HBSS alone was added to the bath of cells at t =120 s. MFAP5 significantly increases the slope of regression line compared with that of HBSS in both cell lines ( P <0.05; two-tailed Student’s t -test). N =number of cells used for the normalized time course. Full size image Since calcium mobilization is linked with increased cell traction force and with cell motility [9] , [10] , we used traction force microscopy to evaluate MFAP5’s effects on changes in cancer cells’ traction force. RecMFAP5 exposure induced an amplitude increase and cell traction force redistribution in A224 and ALST cells ( Fig. 5d,e ), suggesting that directional traction force induction is the physical mechanism of MFAP5-enhanced cell motility and invasion potential. Furthermore, TNNC1 silencing abrogated the amplitude increase in traction force induced by MFAP5 ( Supplementary Fig. 3D ), demonstrating that TNNC1 is the key molecule involved in traction force induction by MFAP5. MFAP5 induces TNNC1 expression via the FAK/CREB signalling Western blot analysis of the key signalling molecules implicated in calcium-dependent pathways and TNNC1 transcriptional regulation demonstrated increases in p-FAK (Y861), p-PLC-γ1 (Y783), p-PKCθ (T538), p-ERK1/2 (T202/Y204), p-CREB (S133), total Jun and p-Jun (S63, S73 and S243) expression in MFAP5-treated cells ( Fig. 6a,b ). On the basis of our results, we hypothesized that binding of MFAP5 to αVβ3 integrin activates FAK. FAK activation activates PLC-γ1 and PKCθ, which regulate Ca 2+ influx. Ca 2+ mobilization leads to ERK1/2 phosphorylation and subsequent CREB activation. Translocation of activated CREB to the nucleus leads to c-Jun transcription via binding of activated CREB to cAMP-response element (CRE) in the c-Jun promoter, which then upregulates TNNC1 expression. Increased TNNC1 protein expression thereby enhances stress fibre formation and cell motility ( Fig. 6c ). 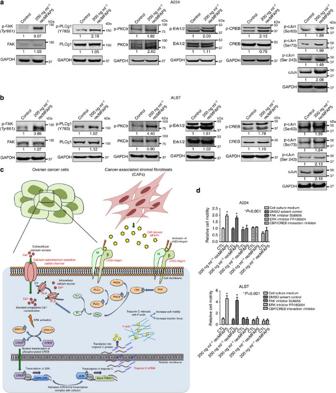Figure 6: Western blot analysis of the key signalling molecules implicated in calcium-dependent pathways and TNNC1 transcriptional regulation. Western blot analyses on proteins isolated from MFAP5-treated A224 and ALST ovarian cancer cells showed that (a) treatment of exogenous MFAP5 increased p-FAK (Y861), p-PLC-γ1 (Y783), p-PKCθ (T538), p-ERK1/2 (T202/Y204), p-CREB (S133), total Jun and p-Jun (S63, S73 and S243) expressions in A224 ovarian cancer cells. (b) Treatment of exogenous MFAP5 increased p-FAK (Y861), p-PLC-γ1 (Y783), p-PKCθ (T538), p-ERK1/2 (T202/Y204), p-CREB (S133), total Jun and p-Jun (S63, S73 and S243) expressions in ALST ovarian cancer cells. Relative normalized protein expression levels with respect to the corresponding control were presented. (c) A graphical summary of the molecular signalling events involved in MFAP5-mediated ovarian cancer cell motility and invasiveness. (d) The presences of FAK, ERK or CBP/CREB interaction inhibitors abrogated the motility-promoting effects of MFAP5 in both A224 and ALST ovarian cancer cells (mean±s.d. of three independent experiments;P<0.001; two-tailed Student’st-test). Figure 6: Western blot analysis of the key signalling molecules implicated in calcium-dependent pathways and TNNC1 transcriptional regulation. Western blot analyses on proteins isolated from MFAP5-treated A224 and ALST ovarian cancer cells showed that ( a ) treatment of exogenous MFAP5 increased p-FAK (Y861), p-PLC-γ1 (Y783), p-PKCθ (T538), p-ERK1/2 (T202/Y204), p-CREB (S133), total Jun and p-Jun (S63, S73 and S243) expressions in A224 ovarian cancer cells. ( b ) Treatment of exogenous MFAP5 increased p-FAK (Y861), p-PLC-γ1 (Y783), p-PKCθ (T538), p-ERK1/2 (T202/Y204), p-CREB (S133), total Jun and p-Jun (S63, S73 and S243) expressions in ALST ovarian cancer cells. Relative normalized protein expression levels with respect to the corresponding control were presented. ( c ) A graphical summary of the molecular signalling events involved in MFAP5-mediated ovarian cancer cell motility and invasiveness. ( d ) The presences of FAK, ERK or CBP/CREB interaction inhibitors abrogated the motility-promoting effects of MFAP5 in both A224 and ALST ovarian cancer cells (mean±s.d. of three independent experiments; P <0.001; two-tailed Student’s t -test). Full size image To test the hypothesis, western blot analyses were performed. Pretreatment with an anti-αVβ3 integrin antibody abrogated MFAP5-induced FAK ( Supplementary Figs 6A and 7A ) and PLC-γ1 phosphorylation ( Supplementary Figs 6B and 7B ), suggesting that αVβ3 integrin is responsible for MFAP5-induced FAK and PLC-γ1 phosphorylation. Previous studies showed that PLC-γ1 phosphorylation is stimulated by both αVβ3 engagement and the formation of the FAK/αVβ3 complex [11] , [12] . We therefore treated cancer cells with an FAK inhibitor to determine whether MFAP5-induced PLC-γ1 phosphorylation is FAK-dependent. The results demonstrated that phosphorylation of p-PLC-γ1 was attenuated in FAK inhibitor-pretreated cells ( Supplementary Figs 6C and 7C ), suggesting that MFAP5-induced pPLC-γ1 phosphorylation is FAK-dependent. Next, we sought to determine whether Ca 2+ mobilization in MFAP5-treated ovarian cancer cells is dependent on p-FAK-mediated PLC-γ1 and PKCθ phosphorylation. Previous studies demonstrated that p-FAK induces PKCθ phosphorylation by activating PLC-γ1 (ref. 13 ). Activated PLC-γ1 increases hydrolysis of intracellular phosphatidylinositol-4,5-bisphosphate to form two products: IP 3 and DAG. IP 3 induces endogenous Ca 2+ release from the endoplasmic reticulum via IP 3 receptors, whereas DAG induces PKCθ phosphorylation and activation. Furthermore, p-PKCθ directly mobilizes Ca 2+ (refs 14 , 15 ). To determine whether PKCθ activation is mediated by p-FAK in MFAP5-treated ovarian cancer cells, western blot analysis of p-PKCθ was performed. The level of p-PKCθ expression increased in MFAP5-treated cells only in the absence of the FAK inhibitor described above ( Supplementary Figs 6D and 7D ). To determine whether the Ca 2+ mobilization observed in MFAP5-treated cells was mediated by PKCθ activation, cells were treated with MFAP5 with or without a PKCθ inhibitor. The PKCθ inhibitor decreased but did not eliminate Ca 2+ mobilization ( Supplementary Fig. 5F ), suggesting that Ca 2+ mobilization is mediated only in part by PKCθ activation. To determine whether PLC activation is involved in Ca 2+ mobilization, we studied the effect of PLC inhibitor U73122 on Ca 2+ mobilization in MFAP5-treated ovarian cancer cells. PLC inhibition effectively suppressed Ca 2+ mobilization ( Supplementary Fig. 5G ), suggesting that PLC activation is the major signalling event involved in MFAP5-mediated Ca 2+ mobilization. However, western blot analysis revealed that PLC inhibitor abolished phosphorylation of PKCθ, and PKCθ inhibitor abolished phosphorylation of PLC-γ1 ( Supplementary Figs 6E,F and 7E,F ), indicating that PLC and PKC are activated interdependently and affect Ca 2+ mobilization in MFAP5-treated cancer cells. To determine whether MFAP5-induced Ca 2+ mobilization activates FAK via a feedback loop, we evaluated the effect of the Ca 2+ chelator BAPTA/AM on MFAP5-induced FAK phosphorylation. We found that MFAP5-induced FAK phosphorylation was abrogated in BAPTA/AM-loaded cells, suggesting that this phosphorylation is Ca 2+ -dependent ( Supplementary Figs 6G and 7G ). Further experiments showed that phosphorylation of ERK1/2 and CREB induced by recMFAP5 was attenuated in cells preloaded with Ca 2+ chelator BAPTA/AM ( Supplementary Figs 6H,I and 7H,I ), and in cells pretreated with PKCθ inhibitor, and PLC inhibitor U73122 ( Supplementary Figs 6J,K and 7J,K ). This suggested that MFAP5-induced ERK and CREB activation is calcium-dependent and is mediated by αVβ3 integrin/FAK/PKCθ- and αVβ3 integrin/FAK/PLCδ activation. CREB is known to be activated by ERK [16] . To determine whether MFAP5 activates CREB via ERK, the effect of an ERK1/2 inhibitor on MFAP5-induced CREB activation was evaluated. Pretreatment of ovarian cancer cells with the ERK1/2 inhibitor abolished the upregulation of p-CREB expression, suggesting that MFAP5 activates CREB via ERK ( Supplementary Figs 6L and 7L ). CREB, together with co-activators, contributes to target gene transcription in response to Ca 2+ and via binding to the CRE. Our data demonstrated upregulation of expression of c-Jun, which contains a CRE in its promoter, in MFAP5-treated cells. In addition, promoter analysis revealed that the TNNC1 promoter consisted of potential AP-1-binding sites ( Supplementary Fig. 8 ), suggesting that transcriptional upregulation of TNNC1 expression is mediated by CREB-mediated c-Jun expression. To verify this, we evaluated the effects of CBP/CREB interaction inhibitor and c-Jun inhibitor SP600125 on MFAP5-treated cells. Results demonstrated that CBP/CREB interaction inhibitor attenuated the upregulation of p-c-Jun ( Supplementary Figs 6M and 7M ), while SP600125 abrogated the upregulation of TNNC1 ( Supplementary Figs 6N and 7N ). MFAP5-induced TNNC1 mRNA expression was abrogated in BAPTA/AM, CBP/CREB interaction inhibitor and c-Jun inhibitor-pretreated cells ( Fig. 7a ). These data confirmed that upregulation of TNNC1 expression induced by MFAP5 is calcium-dependent and mediated via upregulation of c-Jun expression by CREB activation. 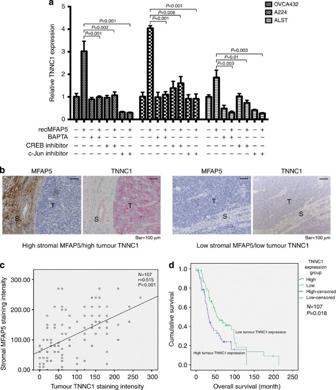Figure 7: Correlation between tumour TNNC1 and stromal MFAP5 expression in human HGSC samples revealed the clinical relevance of TNNC1 to ovarian cancer patient survival. (a) Abrogation of MFAP5-induced increase inTNNC1mRNA expression in A224, ALST and OVCA432 cells after pretreatment with the cell-permeant calcium chelator BAPTA/AM, a CBP/CREB inhibitor or a c-Jun inhibitor (mean±s.d. of three independent experiments; two-tailed Student’st-test). (b) Immunolocalization of TNNC1 and MFAP5 in advanced-stage HGSC tumour sections demonstrating a positive correlation between high stromal MFAP5 and high tumour TNNC1 expression. S, stroma; T, tumour. Bar=100 μm. (c) Positive correlation between stromal MFAP5 expression and tumour TNNC1 expression in HGSC tumours (N=107;r=0.515;P<0.001; Spearman’s Correlation). (d) Kaplan–Meier analysis of the clinical significance of tumour TNNC1 expression with 107 FFPE tumour samples obtained from HGSC patients. Low tumour TNNC1 expression was significantly correlated with improved overall patient survival (N=107;P=0.018; log-rank test). Figure 7: Correlation between tumour TNNC1 and stromal MFAP5 expression in human HGSC samples revealed the clinical relevance of TNNC1 to ovarian cancer patient survival. ( a ) Abrogation of MFAP5-induced increase in TNNC1 mRNA expression in A224, ALST and OVCA432 cells after pretreatment with the cell-permeant calcium chelator BAPTA/AM, a CBP/CREB inhibitor or a c-Jun inhibitor (mean±s.d. of three independent experiments; two-tailed Student’s t -test). ( b ) Immunolocalization of TNNC1 and MFAP5 in advanced-stage HGSC tumour sections demonstrating a positive correlation between high stromal MFAP5 and high tumour TNNC1 expression. S, stroma; T, tumour. Bar=100 μm. ( c ) Positive correlation between stromal MFAP5 expression and tumour TNNC1 expression in HGSC tumours ( N =107; r =0.515; P <0.001; Spearman’s Correlation). ( d ) Kaplan–Meier analysis of the clinical significance of tumour TNNC1 expression with 107 FFPE tumour samples obtained from HGSC patients. Low tumour TNNC1 expression was significantly correlated with improved overall patient survival ( N =107; P =0.018; log-rank test). Full size image To validate the activation of ERK signalling and upregulation of TNNC1 by MFAP5 in vivo , immunostaining of p-ERK1/2 and TNNC1 was performed on paraffin-embedded sections of Matrigel plugs from the previously described animal study. We observed higher p-ERK1/2 and TNNC1 expression in cancer cells in the Matrigel plugs embedded with MFAP5-overexpressing fibroblasts than in cells in the control Matrigel plugs ( Fig. 2h,i ). Following delineation of the underlying signalling mechanism of MFAP5-mediated cell motility, to further demonstrate that the tumour-supportive effects of MFAP5 are dependent on an intact FAK/ERK/CREB/TNNC1 signalling pathway in the cancer cells, we performed cell motility assays on MFAP5-treated ovarian cancer cells in the presence or absence of pathway inhibitors. While both MFAP5 treatment alone and MFAP5 treatment in the presence of DMSO solvent control enhanced motility of A224 and ALST ovarian cancer cells, pretreatment of cancer cells with a FAK inhibitor, ERK inhibitor or CBP/CREB interaction inhibitor abrogated the motility-promoting effects of MFAP5 ( Fig. 6d ). Taken together, with the findings that TNNC1 silencing ( Fig. 4d ) and calcium depletion ( Fig. 5a ) markedly suppressed MFAP5-induced cell motility, these data suggested that MFAP5-induced cancer cell motility is mediated via an intact calcium-dependent FAK/ERK/CREB/TNNC1 signalling pathway in ovarian cancer cells. Clinical relevance of tumour TNNC1 expression The relationship between tumour TNNC1 and stromal MFAP5 expression in 107 HGSC tumour samples was evaluated using immunohistochemistry ( Fig. 7b ) and a significant positive correlation between tumour TNNC1 and stromal MFAP5 expression ( r =0.515, P <0.001) was observed ( Fig. 7c ). Furthermore, Kaplan–Meier analysis revealed that low tumour TNNC1 expression was significantly associated with an improved survival ( P =0.018; log-rank test; Fig. 7d ). Cox regression analysis adjusted for age and debulking status (hazard ratio: 1.705; P =0.029) confirmed the prognostic significance of tumour TNNC1 expression. In the tumour microenvironment, the dynamic and reciprocal interactions among cells, the extracellular matrix and soluble molecules dictate tumour progression [17] . CAFs have higher proliferation rates than do normal fibroblasts and often have enhanced production of collagen, hyaluronate and epithelial growth factors [18] , [19] . Researchers have demonstrated that CAFs that secrete chemokines at elevated levels promote the initiation and development of ovarian cancer [20] . Furthermore, the complex stromal microenvironment has made therapeutic elimination of cancer impossible for decades [2] . In the present study, we identified CAF-derived MFAP5 as a prognostic marker for poor survival. MFAP5 is involved in elastic microfibril assembly and modulates endothelial cell behaviour [21] , [22] . Focusing on the epithelial component of HGSC, our group previously identified MFAP5 as a survival-associated target in HGSC. We observed MFAP5 amplification and overexpression in a small percentage of advanced HGSC cases [6] . In addition, we found that ovarian cancer-derived MFAP5 promoted tumour cell survival and stimulated endothelial cell motility and survival via the αVβ3 integrin receptor. However, to our surprise, transcriptome profiling of the stromal component of HGSCs revealed that CAFs had much higher expression of MFAP5 mRNA than did the normal ovarian stroma and epithelial components of ovarian tissue. In addition, immunolocalization of MFAP5 using a newly developed antibody confirmed that ovarian cancer stroma indeed has markedly higher levels of MFAP5 expression than did the epithelial component, which we did not observed in our previous study. This discrepancy is likely a result of the fact that stromal MFAP5 may be crosslinked with other proteins in the stroma more tightly during the formalin fixation process and requires higher antigen retrieval temperatures to re-expose the epitope recognized by the antibodies that have higher affinity to MFAP5. To strengthen the significance of CAFs as sources of MFAP5 in the tumour microenvironment, western blot analyses on samples from immortalized CAFs, primary CAFS as well as HGSG cancer cell lines were also performed. While some HGSC cell lines express a detectable amount of MFAP5, our data confirmed that CAFs are the major sources of MFAP5 in the ovarian tumour microenvironment. In addition, in cases in which tumour cells have low levels of MFAP5 expression but high levels of stromal MFAP5 expression, stromal MFAP5 secreted from CAFs may exert a paracrine effect on ovarian cancer cells and contribute to ovarian tumour progression. Our correlation studies demonstrated that epithelial and stromal MFAP5 expressions in tumour tissue were significantly associated with each other ( Supplementary Fig. 9 ). Therefore, it is not a surprise to find out that high levels of stromal MFAP5 expression, similar to the epithelial MFAP5 expression as reported in the previous study, were also significantly associated with poor patient survival. The significant association between stromal and epithelial MFAP5 expression suggests that MFAP5 is regulated by certain tumour microenvironmental cues in the same manner. However, the molecular mechanism by which stromal MFAP5 is expressed at high levels remains to be elucidated. Our in vitro data demonstrated a significant increase in ovarian cancer cell motility and invasion potential but not cell proliferation after treatment with recombinant MFAP5 protein ( Supplementary Fig. 3E,F ). To evaluate the role of CAF-derived MFAP5 on cell migration and invasion potentials in vivo , we developed a new model that allows for the interaction between MFAP5-secreting CAFs and cancer cells in the intraperitoneal microenvironment. In this model, a Matrigel plug embedded with MFAP5-secreting CAFs recapitulates a substratum through which cancer cells invade MFAP5-expressing CAFs in the tumour. The results of our study of this model demonstrated that Matrigel plugs with MFAP5 represent a better soil for cancer cells to invade. Effects of MFAP5 on cancer metastasis was further evaluated by injecting MFAP5 -specific siRNA-encapsulated nanoparticles into an orthotopic model in which ovarian cancer cells were injected into the ovary. This significantly decreased in the number of metastatic nodules and the organs involved in MFAP5 siRNA-treated mice compared with the control, suggesting the therapeutic potential of targeting stromal MFAP5 as a new treatment modality, which may improve survival. Our findings demonstrated that Ca 2+ mobilization is essential for MFAP5’s effects on ovarian cancer cell motility and invasion potential. Ca 2+ plays a multifunctional role in cell migration, including cytoskeleton redistribution and focal adhesion relocation [23] , [24] , [25] , [26] . Five major classes of membrane Ca 2+ -permeable channels are known to be differentially expressed in various cell types, and the authors recently identified additional channels [27] , [28] . The present study demonstrated that treatment with an L-type Ca 2+ channel blocker attenuated MFAP5-induced calcium influx but did not abolish this effect, whereas treatment with an L-type Ca 2+ channel opener successfully stimulated calcium entry in ALST cells, suggesting that MFAP5 triggers exogenous Ca 2+ entry into ALST cells via the L-type voltage-gated channel, although other channels may be involved. Treatment with an IP 3 receptor inhibitor but not a ryanodine receptor blocker attenuated MFAP5-induced calcium mobilization, suggesting that MFAP5 induces calcium release via the IP 3 receptor instead of the ryanodine receptor. This was supported by our finding that MFAP5 activates PLC-γ1 phosphorylation, which may lead to hydrolysis of intracellular phosphatidylinositol-4,5-bisphosphate to IP 3 and DAG. IP 3 binds to its receptor, causing Ca 2+ release from the endoplasmic reticulum. Calcium is a prominent regulator of cell migration, exerting multiple effects on the contractility of the actin cytoskeleton [10] , [29] . Our findings, of abrogation of which MFAP5-induced actin rearrangement, stress fibre condensation, and traction force by BAPTA/AM, suggest calcium-dependent actin reorganization, together with increased traction force modulate MFAP5’s motility and invasion promoting effects. TNNC1 contains a calcium-binding subunit and facilitates the interaction between actin and myosin in muscle cells and the formation of stress fibres [30] . Indeed, troponin is expressed not only in striated muscle cells but also in fibroblasts [31] . In nonmuscle cells, TNNC1 may not serve as a structural protein but rather as a regulatory protein for cellular locomotion, cytoplasmic streaming and cytokinesis [30] . In the present study, we demonstrated for the first time that TNNC1 is overexpressed in epithelial ovarian cancer cells and that siRNA silencing of TNNC1 abolishes MFAP5’s stimulatory effect on cancer cells. This is the first study to demonstrate that increased TNNC1 expression modulates epithelial cancer cell motility and invasion potential via cytoskeleton reorganization. In addition, immunolocalization of TNNC1 on HGSC samples demonstrated the positive correlation between cancer cell TNNC1 expression and stromal MFAP5 expression and the association between increased TNNC1 expression and poor survival. These data confirmed that TNNC1 is the effector protein for stromal MFAP5, which can promote cell motility and invasion potential via tumour–stromal crosstalk and subsequently affect clinical outcome. Of note, we observed that TNNC1 silencing did not affect ovarian cancer cell proliferation ( Supplementary Fig. 3G,H ), suggesting that the effect of MFAP5 on tumour growth we observed in vivo is indirect, most likely via its effect on other cell types in the microenvironment. In fact, our group has demonstrated a correlation between increased MFAP5 expression and microvessel density [6] , suggesting that the proangiogenic role of MFAP5 may lead to increased tumour growth in vivo . In conclusion, we found that CAF-derived MFAP5 modulated ovarian cancer cell motility and invasion potential via the calcium-dependent FAK/CREB/TNNC1 signalling pathway. Targeting stromal MFAP5 with siRNA-encapsulated CH-NPs markedly decreased tumour growth and metastasis in vivo , suggesting that it is a new treatment modality for ovarian cancer. Microdissection and profiling of tissue samples Ovarian tissue samples were obtained from the ovarian cancer repository of the Department of Gynecologic Oncology and Reproductive Medicine at The University of Texas MD Anderson Cancer Center under protocols approved by the MD Anderson Institutional Review Board. All tumour samples were obtained from the primary ovarian sites of pretreatment cases. Microdissection was performed as described by Yeung et al . [32] to isolate the stromal and epithelial components of normal and malignant ovarian tissue for RNA extraction. In brief, tissue sections were fixed in 70% ethanol and stained with 1% methyl green to visualize the histologic features. During dissection, areas with immune cell and blood vessel infiltration were excluded to minimize contamination. Purified RNA samples were amplified, labelled and hybridized on GeneChip Human Genome U133 Plus 2.0 microarrays (Affymetrix Inc., Santa Clara, CA, USA) according to the manufacturer’s protocol. After hybridization, arrays were washed and stained using a Fluidics Station 450 and then scanned using a GeneChip Scanner 3000 7G (Affymetrix Inc.). Cell lines and culture conditions Human ovarian adenocarcinoma cell lines A224, ALST (gifts from Dr Michael Birrer’s laboratory at the Massachusetts General Hospital), OVCA432 (gift from Dr Robert Bast’s laboratory at the MD Anderson Cancer Center) and SKOV3ipluc (obtained from American Type Culture Collection) were maintained in RPMI 1640 medium supplemented with 10% fetal bovine serum, 2 mM glutamine and penicillin–streptomycin. The immortalized human NOF line NOF151-hTERT and primary CAF lines were cultured in 1:1 MCDB105/199 medium supplemented with 10% fetal bovine serum, 1 ng ml −1 epidermal growth factor and penicillin–streptomycin. Quantitative real-time RT–PCR analysis The relative expression of each target gene was calculated using the 2 −ΔΔ C t method to average the C t value of the housekeeping gene for a single reference gene value. Pre-designed human MFAP5 (Hs00185803_m1), TNNC1 (Hs00896999_g1), cyclophilin A (Hs99999904_m1) and murine Mfap5 (Mm00489404_m1) TaqMan gene expression assays (Life Technologies Corp., Grand Island, NY, USA) were used in the PCR analysis. Western blot analysis Protein lysates from CAFs, normal fibroblasts and ovarian cancer cells were separated on 10% sodium dodecyl sulfate NuPAGE gels under denaturing conditions and transferred on nitrocellulose membranes using an iBlot Western blotting system (Life Technologies Corp.) before being incubated with primary antibodies. Anti-human MFAP5 (1:1,000; no. HPA010553) was purchased from Sigma-Aldrich Co. (St Louis, MO, USA). An anti-p-FAK antibody (Y861; 1:1,000; no. 44-626G) was purchased from Life Technologies Corp. All other antibodies, including anti-FAK (1:1,000; no. 3285), anti-PLC-γ1 (1:1,000; no. 2822), anti-p-PLC-γ1 (T783; 1:1,000; no. 2821), anti-PKCθ (1:1,000; no. 2059), anti-p-PKCθ (T538; 1:1,000; no. 9377), anti-ERK1/2 (1:1,000; no. 9102), anti-p-ERK1/2 (T202/204; 1:1,000; no. 9101), anti-CREB (1:1,000; no. 9197), anti-p-CREB (S133; 1:1,000; no. 9198), anti-c-Jun (1:1,000; no. 9165) and anti-p-c-Jun (S63, S73 and S243; 1:1,000; no. 2361, no. 9164 and no. 2994, respectively), were purchased from Cell Signaling Technology (Beverly, MA, USA). After being washed with Tris-buffered saline with Tween, the membranes were incubated with a goat anti-rabbit IR dye-conjugated secondary antibody (1:5,000; LI-COR Biosciences, Lincoln, NE, USA). Protein bands were detected using an Odyssey infrared imaging system (LI-COR Biosciences). The ImageJ software programme (National Institutes of Health, Bethesda, MD, USA) was used to quantify band intensities of western blot images. Protein expression levels in terms of band intensities were normalized against protein loading using the housekeeping gene as reference. Relative protein expression levels were presented with respect to their corresponding controls, which had the baseline of 1. The inhibitors used in pathway analyses included a PLC inhibitor (U73122; no. sc-3574), PKCθ pseudosubstrate inhibitor (no. sc-3097) and ERK inhibitor II (FR180204; no. sc-203945), which were purchased from Santa Cruz Biotechnology (Santa Cruz, CA, USA). An FAK inhibitor (SU6656; no. S9692) and a c-Jun inhibitor (no. SP600125) were purchased from Sigma-Aldrich Co., and a CBP/CREB interaction inhibitor (no. 217505) was purchased from EMD Millipore Corp. (Billerica, MA, USA). Original images for essential blots are supplied as Supplementary Information ( Supplementary Figs 10 and 11 ). Immunohistochemical analysis Immunolocalization of MFAP5 and TNNC1 was performed using 130 and 107 FFPE ovarian tumour sections, respectively, obtained from HGSC patients. Slides containing the sections were stained with commercially available anti-MFAP5 (1:500; no. HPA010553) and anti-TNNC1 (1:100; no. WH0007134M1) antibodies (Sigma-Aldrich Co.). Target protein expression was visualized using a Betazoid 3,3′-diaminobenzidine or Warp Red chromogen kit (Biocare Medical, Concord, CA, USA). To quantify target protein expression in the FFPE sections, slides were scored according to the staining intensity and percentage of MFAP5- and TNNC1-positive cells. To quantify stromal MFAP5 expression, the expression scores were calculated by multiplying the staining intensity (range, 0–3) by the percentage of stroma with MFAP5-positive staining. TNNC1 tumour expression scores were calculated as the products of staining intensity and percentage of TNNC1-positive staining. Stromal MFAP5-stimulated motility of ovarian cancer cells CAF793092 cells were seeded on a 24-well plate at a density of 5 × 10 4 cells per well. The culture medium was then removed from the plate, and cells were washed with PBS the next day. Serum-free M105/199 media supplemented with 1 ng ml −1 epidermal growth factor and 10 μg ml −1 control IgG or anti-MFAP5, anti-αVβ3 or anti-α5 antibodies were added to the wells. Seventy-two hours later, 5 × 10 4 A224 or ALST cells were seeded on each 8-μm insert (BD Biosciences, San Jose, MA, USA) in the serum-free medium and co-cultured with CAFs. After 15 h of incubation, the cells were stained with calcein AM (Life Technologies Corp.), and nonmigrating cells in the upper surface of the insert were removed. The migrated cells in each chamber were counted by obtaining images of the stained cells in nine random fields of view per membrane using a fluorescent microscope and quantified using the Image-Pro Plus 7.0 software programme (Media Cybernetics Inc., Rockville, MD, USA). Recombinant MFAP5-increased ovarian cancer cell motility OVCA432 cells were seeded on chamber slides in 10% serum RPMI medium. After they attached to the slides, they were washed with PBS, and serum-free RPMI medium with or without 500 ng ml −1 recMFAP5 was added to the wells. The cells were then placed in an imaging chamber maintained at 37 °C and supplemented with 5% CO 2 . Cell images were taken every 15 min for 48 h using confocal microscopy and the resulting series of images was imported into the MetaMorph software programme to track the movement of individual cells. To confirm exogenous MFAP5’s effects on ovarian cancer cell motility, a motility assay was performed using a Boyden chamber with two additional ovarian cancer cell lines: A224 and ALST. Serum-free RPMI medium alone or with 500 ng ml −1 recMFAP5 was incubated with 10 μg ml −1 control IgG or anti-MFAP5, anti-αVβ3 or anti-α5 antibodies for 1 h in the wells of 24-well plates. Monoclonal anti-αVβ3 antibody (no. MAB1976Z) was purchased from EMD Millipore Corp., and an anti-α5 antibody (no. 555615) was purchased from BD Bioscience. A224 or ALST cells (5 × 10 4 ) were then seeded on each 8-μm insert (BD Biosciences) in serum-free medium and incubated for 15 h. Cells were stained with calcein AM (Life Technologies Corp.), and nonmigrating cells were removed from the upper surface of the inserts. The migrated cells in each chamber were counted by obtaining images of stained cells in nine random fields of view per membrane using a fluorescent microscope and quantified using the Image-Pro Plus 7.0 software programme (Media Cybernetics Inc.). To evaluate the role of calcium and TNNC1 in cell motility induced by MFAP5, ovarian cancer cells were pretreated with the cell-permeant calcium chelator BAPTA/AM (B-6769; Life Technologies Corp.) at a concentration of 10 μM for 1 h or transfected with efficiency-evaluated TNNC1 -specific siRNA (Hs00896999_g1; Life Technologies Corp.; Supplementary Fig. 3B,C ) before performing the motility assay with recMFAP5. MFAP5-stimulated ovarian cancer cell invasion The invasion potential of ovarian cancer cells treated with recMFAP5 was evaluated using a Matrigel invasion assay with a BD BioCoat Matrigel invasion chamber (BD Biosciences) according to the manufacturer’s protocol. In brief, 3 × 10 4 A224 or ALST cells were seeded on an 8-μm BD BioCoat Matrigel invasion chamber in a serum-free medium and inserted into a BD Falcon TC companion plate with or without 200 ng ml −1 recMFAP5. The cells were incubated in a humidified tissue culture incubator at 37 °C in a 5% CO 2 atmosphere for 15 h. Cells were then stained with calcein AM, and non-invading cells were removed from the upper surface of the invasion chambers. Counting of the invaded cells was facilitated by photographing the membrane under a fluorescent microscope, and the numbers of invaded cells were analysed using the Image-Pro Plus 7.0 software programme (Media Cybernetics Inc.). Derivation of MFAP5-overexpressing NOFs The telomerase-immortalized human NOF line NOF151-hTERT was transduced with lentiviruses packaged with an open reading frame lentiviral expression clone (no. EX-D0360-Lv105; GeneCopoeia, Rockville, MD, USA) for 48 h. Transduced cells were selected using complete medium supplemented with puromycin at a working concentration of 1 μg ml −1 for 5 days. MFAP5 expression in the NOFs was measured using western blot analysis, in which the lysate and conditioned medium from the resultant NOF line NOF151-LvMFAP5 were compared with those from the mock-transduced control line. A proliferation assay was performed using an xCELLigence system (Roche Applied Bioscience, Indianapolis, IN, USA) to ensure that the NOF151-LvMFAP5 and NOF151-hTERT cells had similar growth rates. MFAP5 stimulated cancer cell migration and invasion in vivo Normal parental NOF151 cells (5 × 10 4 ) or MFAP5-overexpressing NOF151 cells (NOF151-LvMFAP5) resuspended in one part of PBS were mixed with two parts of Matrigel, and the mixture was injected into the intraperitoneal cavity of anaesthetised female nude mice at the age of 6 weeks. The mixture (500 μl) was injected into each animal and allowed to warm to body temperature to form a Matrigel plug attached to the peritoneal wall. The next day, 1 million A224 or OVCA432 cells were injected intraperitoneally into the mice. Matrigel plugs were harvested from A224- and OVCA432-injected mice at 48 and 72 h post cancer cell injection, respectively. The resected plugs were fixed in formalin and processed for histological evaluation. The described animal procedures have been reviewed and approved by the institutional animal care and use committee of the MD Anderson Cancer Center. In vivo Mfap5 silencing-reduced tumour progression Luciferase-labelled OVCA432ip ovarian cancer cells were suspended in 50 μl of Hanks balanced salt solution (HBSS) and injected directly into the left ovary of anaesthetised female nude mice at the age of 6 weeks through a 1.5-cm intraperitoneal incision. One week after cell injection, CH-NPs packaged with Mfap5 -targeting siRNA or nontargeting siRNA were injected intravenously into nude mice twice a week for a total of 6 weeks. Seven weeks after initial injection, tumour volume of each treatment group was quantified by the IVIS-200 bioluminescence and fluorescence imaging system (Caliper Life Sciences Inc., Hopkinton, MA, USA). At week 8, the animals were killed and necropsy was performed. The number, weight and location of individual tumour nodules were identified and recorded. Tumour tissues were fixed in formalin and processed for histological evaluation. The described animal procedures have been reviewed and approved by the institutional animal care and use committee of the MD Anderson Cancer Center. MFAP5 activated signalling in cancer cells RNAs were isolated from OVCA432 cells and treated with PBS or 200 ng ml −1 recMFAP5. Total RNA (100 ng) from each group were used to generate biotin-labelled aRNA and then subjected to whole-genome transcriptome profiling using GeneChip Human Genome U133 Plus 2.0 microarrays (Affymetrix Inc.). Differentially expressed genes, which were expressed at levels more than 1.5-fold higher than those of the corresponding controls P <0.05, were selected for further analyses using the Ingenuity Pathway Analysis software programme. MFAP5-stimulated calcium-dependent F-actin rearrangement A224 and ALST cells were seeded on Lab-Tek chamber slides (Thermo Fisher Scientific, Pittsburgh, PA, USA), and serum-free medium was added to the wells the next day to fast the cells overnight. Cells were then treated with fresh serum-free medium supplemented with PBS or 200 ng ml −1 recMFAP5 for 24 h. After incubation, cells were fixed with 3.7% formaldehyde and stained with Alexa Fluor 594 phalloidin (Life Technologies Corp.) according to the manufacturer’s instructions. Fluorescent microscopy was used to evaluate the F-actin rearrangement in cells stimulated by MFAP5. To evaluate the role of calcium and TNNC1 in F-actin reorganization induced by MFAP5, ovarian cancer cells were pretreated with the cell-permeant calcium chelator BAPTA/AM (B-6769; Life Technologies Corp.) for 1 h and transfected with TNNC1 -specific siRNA, respectively, before MFAP5 treatment and staining with Alexa Fluor 594 phalloidin. Protein fractionation and western blot analysis of TNNC1 Knockdown of TNNC1 protein expression in A224 and ALST cells by siRNA transfection was confirmed using western blot analysis. Before this analysis, cell pellets were collected from non-target scrambled and TNNC1 -targeting siRNA-transfected A224 and ALST cells, and cytoplasmic protein fractions of the lysates were isolated using the NE-PER nuclear and cytoplasmic extraction reagents (Thermo Fisher Scientific Inc., Waltham, MA, USA) according to the manufacturer’s protocol. A polyclonal rabbit anti-human TNNC1 antibody (1:500; 13504-1-AP; Proteintech, Chicago, IL, USA) was used to determine TNNC1 expression levels in the cytoplasmic protein factions via western blot analysis. Traction force microscopy The cell traction force exerted on a flexible substrate impregnated with fluorescent microspheres by A224 or ALST cells growing on the substrate was determined according to measured substrate displacements using the LIBTRC analysis library developed by Micah Dembo of the Boston University [33] , [34] , [35] . In brief, polyacrylamide gel (5% acrylamide and 0.1% Bis-acrylamide, 75-μm thick; Young’s modulus=5.8 kN m −2 ) was prepared on glass coverslips with fluorescent microspheres (0.2 μm diameter, yellow-green FluoSpheres; Life Technologies Corp.) impregnated under the top surface. The surface was then coated with 0.2 mg ml −1 collagen type I (BD Bioscience) after photoactivation of the surface molecular linker sulfosuccinimidyl-6-(4′-azido-2′-nitrophenylamino) hexanoate (sulfo-SANPAH; Pierce Chemical, Dallas, TX, USA). Cells were seeded and cultured overnight. To evaluate the effect of exogenous MFAP5 on the traction force exerted by cancer cells on the substratum, cancer cells were treated with exogenous MFAP5 in HBSS and a series of images of a single individual cancer cell was captured during the course of each experiment. A background image of the fluorescent beads was also taken after the cell was removed from the substrate. The LIBTRC library was then used to track the displacement of microspheres and compute the cell traction force. Total traction force (cell surface area × traction force per unit area) was normalized by the total traction force of the same cell before exposure to MFAP5 or HBSS. One cell was studied for each coverslip. All images were collected using a TCS SP5 confocal microscope (Leica Microsystems, Buffalo Grove, IL, USA). [Ca 2+ ] i measurement A224 or ALST cells that grew on collagen-coated Petri dishes with glass bottoms were loaded with Fluo-4 AM in HBSS for 30 min followed by 20 min to de-esterify the dye. Fluo-4 AM was excited at 488 nm, and its emission was collected using a bandpass filter at 522/35 nm. Fluorescent images of the cells were collected using a Leica TCS SP5 confocal microscope at 0.25 Hz. Statistical analysis The SPSS 19 (IBM Corp., Armonk, NY, USA) and Prism 5.0 (GraphPad Software, La Jolla, CA, USA) software programs were used to perform statistical tests. All in vitro experiments were repeated independently in triplicate. A two-tailed Student’s t -test was used to determine differences in the sample means for data with normally distributed means. The Mann–Whitney U -test was used for analysis of nonparametric data. A P -value less than 0.05 was considered statistically significant. How to cite this article: Leung, C. S. et al . Calcium-dependent FAK/CREB/TNNC1 signalling mediates the effect of stromal MFAP5 on ovarian cancer metastatic potential. Nat. Commun. 5:5092 doi: 10.1038/ncomms6092 (2014).